Plasmon-induced photonic and energy-transfer enhancement of solar water splitting by a hematite nanorod array Plasmonic metal nanostructures offer a promising route to improve the solar energy conversion efficiency of semiconductors. Here we show that incorporation of a hematite nanorod array into a plasmonic gold nanohole array pattern significantly improves the photoelectrochemical water splitting performance, leading to an approximately tenfold increase in the photocurrent at a bias of 0.23 V versus Ag|AgCl under simulated solar radiation. Plasmon-induced resonant energy transfer is responsible for enhancement at the energies below the band edge, whereas above the absorption band edge of hematite, the surface plasmon polariton launches a guided wave mode inside the nanorods, with the nanorods acting as miniature optic fibres, enhancing the light absorption. In addition, the intense local plasmonic field can suppress the charge recombination in the hematite nanorod photoanode in a photoelectrochemical cell. Our results may provide a general approach to overcome the low optical absorption and spectral utilization of thin semiconductor nanostructures, while further reducing charge recombination losses. Solar energy conversion is a promising way to provide a sustainable energy source to meet the steadily increasing energy demand. Solar energy can be converted and stored in chemical fuels with a photoelectrochemical cell (PEC) by splitting water or reducing CO 2 (refs 1 , 2 , 3 , 4 , 5 , 6 , 7 , 8 ). The key to the success of solar fuel production with PECs is the development of high-performance photoelectrodes. However, the poor performance of current semiconductor photoelectrodes is dictated by several constraints such as limited light-absorption wavelength range, low-efficiency charge separation and/or high charge recombination rate. For example, TiO 2 , which serves as the benchmark of photoelectrode materials, is able to only absorb ultraviolet light due to its wide band gap (3.26 eV for anatase TiO 2 ) [9] , [10] . Hematite (α-Fe 2 O 3 ) is another potential photoelectrode material, which is stable, non-toxic, inexpensive and earth-abundant. Although it has an appealing band gap (1.9–2.2 eV), its application in the photoelectrode is hindered by several shortcomings as follows [5] , [6] , [7] , [11] , [12] : a short hole diffusion length (2–4 nm) compared with its light penetration depth (~120 nm), short lifetime of charge carriers (<10 ps) and poor mobility of charge carriers (<0.2 cm 2 V −1 s −1 ). Hematite can be engineered into a nanostructure to reduce the charge-carrier diffusion distance to the electrode/electrolyte interface, and to combat the short carrier lifetime. However, the trade-off is that to satisfy the diffusion length, the structure must be much smaller than the optical absorption depth, limiting the amount of light collected [13] , [14] , [15] , [16] , [17] , [18] , [19] . In fact, no single material can meet all the requirements of an ideal photoelectrode in PECs so far. An effective approach for overcoming this trade-off is integrating a plasmonic metal nanostructure with a semiconductor to reclaim the light no longer absorbed [20] , [21] , [22] , [23] , [24] , [25] , [26] , [27] . Surface plasmon resonance (SPR) exists in two distinct forms: surface plasmon polaritons (SPP) and localized SPR (LSPR) [21] , [23] , [28] . SPP, or propagating surface plasmons, are travelling charge oscillations resonantly excited on the surface of thin metal films, whereas LSPR is the stationary, non-propagating collective oscillation of the surface electrons in metal nanostructures. Utilization of SPP and LSPR in plasmonic nanostructures can improve the solar energy conversion efficiency of semiconductors via two pathways [28] : photonic enhancement and plasmonic energy-transfer enhancement. For large or patterned plasmonic nanostructures, the incident light is efficiently scattered multiple times, increasing the optical path length and the light absorption in thin semiconductor layers [20] , [21] , [22] , [23] , [24] , [25] , [26] . This is referred to as photonic enhancement (or light trapping) [21] , [26] , [28] , which contributes to enhancement at the energies above the band gap of a semiconductor. Alternatively, if the local field enhancement and absorption cross-section is large, LSPR can induce charge separation in the semiconductor by absorbing light at the energies below the band gap and transferring the energy to the semiconductor [27] , [28] , [29] , [30] , [31] , [32] , [33] , [34] . The LSPR-induced charge separation can occur by transferring the energy contained in the oscillating electrons or local plasmonic field from the metal to the semiconductor via (i) direct electron transfer (DET) [29] , [30] and/or (ii) plasmon-induced resonant energy transfer (PIRET) [31] . This is referred to as plasmonic energy-transfer enhancement [28] and is strong in small metal nanoparticles with small scattering cross-sections. In the DET process, the semiconductor must be in intimate contact with the plasmonic metal, allowing the LSPR-excited hot electrons to overcome the Schottky barrier between the metal and semiconductor [29] , [30] , [31] , [32] . The efficiency of DET is determined by the relative energy of hot electrons in the metal to the height of the Schottky barrier at the interface. In contrast, PIRET proceeds non-radiatively based on the near-field dipole–dipole interaction between the plasmonic metal and the semiconductor [31] , [32] . PIRET does not require direct contact or band alignment; instead, the efficiency is determined by the spectral overlap between the semiconductor’s absorption band edge and the LSPR absorbance [31] , [32] . PIRET allows the light absorption and the charge separation in a semiconductor at the energies below the band edge. As mentioned above, solar energy collection can be enhanced by plasmonic nanostructures via photonic or/and plasmonic energy-transfer enhancement [28] . Unfortunately, because of the geometric trade-off between the scattering and absorption efficiency, either the photonic or the plasmonic energy-transfer enhancement is currently utilized separately only in a narrow spectral region of solar spectrum [26] , [27] . In many cases, although plasmonic nanostructures can be optimized to strongly absorb incident solar light, the collected energy cannot be effectively transferred to the semiconductor due to weak coupling between the plasmonic nanostructure and the semiconductor. To date, it remains a significant challenge to develop efficient plasmonic metal–semiconductor heterostructures that can fully utilize the plasmonic effects for enhancement of the light absorption and charge-separation processes in semiconductors. This report shows that the trade-off between photonic and plasmonic energy-transfer enhancement can be overcome by utilizing both SPP and LSPR to enhance the PEC performance in a wide range of the solar spectrum via a unique heterostructure, which consists of a hematite nanorod array grown on a plasmonic gold nanohole array pattern. The long-range ordered gold nanohole array supports both propagating (SPP) and localized (LSPR) plasmon modes, which is the key to overcoming the scattering/absorption trade-off. On a local scale, the nanohole in the metal film leads to a LSPR mode with energy below the band gap of hematite [35] , [36] , which increases the spectral coverage through PIRET. The long-range order of the nanohole array creates a grating, giving incident light sufficient momentum to excite a SPP mode at the energies above the band edge of hematite. As is well known, the SPP leads to extraordinary optical transmission through the nanohole array at the resonant wavelengths [37] , [38] , [39] . As the nanohole array is filled with the hematite nanorods, the extraordinary optical transmission launches a guided mode inside the nanorod similar to an optical fibre, further enhancing light absorption in hematite. In addition, the present work shows that the intense local plasmonic field at the metal/hematite interface can prolong the charge-carrier lifetime in hematite. In short, the hematite–Au heterostructure not only reduces the charge recombination rate but also enables both photonic and plasmonic energy-transfer enhancement in a wide ultraviolet–near-infrared spectral region. Microstructure The long-range ordered plasmonic Au nanohole array pattern was fabricated using nanosphere lithography on a fluorine-doped tin oxide (FTO) substrate (see Supplementary Fig. S1 ) [40] , [41] , [42] . The Au nanoholes were 85 nm high and 350 nm in diameter ( Fig. 1b ). The centre-to-centre distance between adjacent holes was around 490 nm. The hole width, pitch and the Au film thickness were chosen to enable the SPP and LSPR modes at the wavelengths below and above the band gap of hematite, respectively. The hematite nanorods were grown on the Au nanohole array pattern with a hydrothermal method, followed by annealing at 650 °C ( Fig. 1a ) [43] . The hematite nanorods were grown inside the hole regions. Hematite displayed the same nanorod morphology on both the bare FTO and the Au nanohole array pattern ( Fig. 1c and Supplementary Fig. S2 ). Transmission electron microscopy (TEM), higher-resolution TEM and X-ray diffraction confirmed the formation of hematite (see Supplementary Figs S3 and S4 ). 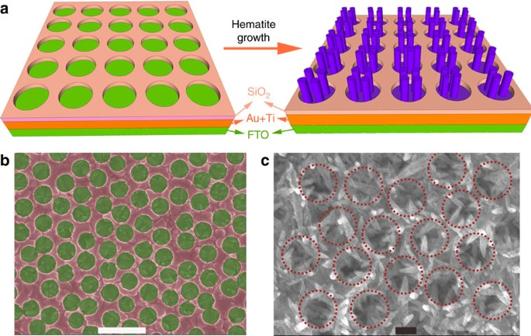Figure 1: Architecture and microstructure of plasmonic photoanode. (a) Scheme for the growth of the hematite nanorod array on the Au nanohole array. (b,c) Scanning electron microscopic images of the Au nanohole array without (b) and with (c) the hematite nanorods. Scale bars, 1 μm (b) and 200 nm (c). Figure 1: Architecture and microstructure of plasmonic photoanode. ( a ) Scheme for the growth of the hematite nanorod array on the Au nanohole array. ( b , c ) Scanning electron microscopic images of the Au nanohole array without ( b ) and with ( c ) the hematite nanorods. Scale bars, 1 μm ( b ) and 200 nm ( c ). Full size image Optical properties The ultraviolet–visible absorption spectrum of the bare Au nanohole array pattern had a strong absorption peak centred at 650 nm and an enhanced transmission peak at 475 nm compared with an unpatterned gold film of the same thickness (see Supplementary Fig. S5 ). The hematite nanorods grown on the bare FTO substrate absorbed light with a tail up to 700 nm. The band gap was determined to be 2.0 eV, using a tangent line to the absorption edge ( Fig. 2a ). The additional exponentially decaying absorption tail was attributed to an Urbach tail formed by defect states in hematite. When the hematite nanorods were grown on the Au nanohole array, an increase in absorption across the entire spectral range was seen compared with hematite on bare FTO. After division of the hematite background from the hematite/nanohole array sample, an absorption band centred at around 650 nm was observed ( Fig. 2b ), which matched the LSPR peak for the bare Au nanohole array pattern. The enhancement factor represents the division of the two ultraviolet–visible spectra (not the percentage change). The high tail after 750 nm is an artefact of the division process due to the low absorption coefficient of hematite at higher wavelengths ( Fig. 2a ). The nanohole array transmission peak centred at 475 nm was not as easily seen in the hematite/nanohole array sample as the absorption peak at 650 nm. However, the absorption was seen to be enhanced proportional to the band edge of hematite ( Fig. 2a ). As the hematite nanorods on the Au nanohole array pattern had lower density when compared with those grown on bare FTO, the SPP must be responsible for the increase in the absorption of light in hematite above the band gap. 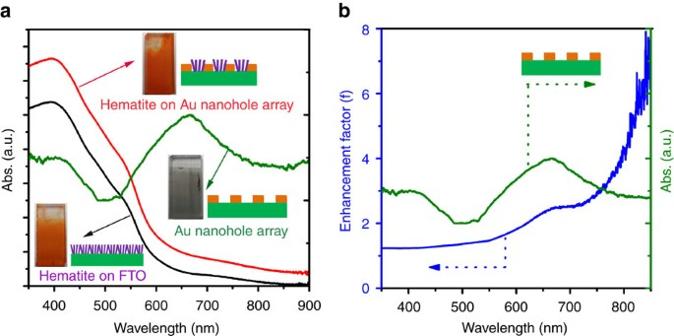Figure 2: Plasmon-enhanced light absorption. (a) Ultraviolet–visible absorption spectra for 150-nm long hematite nanorods on the bare FTO and on the Au nanohole array pattern, respectively. The insets show the corresponding digital pictures of photoanodes. (b) Absorption enhancement for the hematite nanorods on the Au nanohole array pattern with the background (hematite on FTO) subtracted. Figure 2: Plasmon-enhanced light absorption. ( a ) Ultraviolet–visible absorption spectra for 150-nm long hematite nanorods on the bare FTO and on the Au nanohole array pattern, respectively. The insets show the corresponding digital pictures of photoanodes. ( b ) Absorption enhancement for the hematite nanorods on the Au nanohole array pattern with the background (hematite on FTO) subtracted. Full size image Photoelectrochemical performance The PEC performance was measured in 1.0 M NaOH electrolyte using a three-electrode cell for the hematite nanorods on both the bare FTO and the Au nanohole array pattern ( Supplementary Fig. S6 ). For the PEC measurements, the photoanode was backside illuminated by 100 mW cm −2 of simulated solar light from a 300-W Xenon lamp through an AM 1.5G solar simulator filter. The current density in Fig. 3a was calculated based on the whole geometric area of photoanode instead of the effective electro-active area (hole regions) on the photoanode. The photocurrent was significantly enhanced for the 150-nm long hematite nanorods grown on the gold nanohole array pattern when compared with hematite grown on bare FTO ( Fig. 3a ), with an enhancement factor as high as 10 at a bias of 0.23 V (versus Ag|AgCl) under the simulated solar full spectrum. The onset potential of the photocurrent remained the same for the hematite nanorods on both the bare FTO and the Au nanohole array pattern, which indicated that the Au nanohole array pattern had negligible influence on the surface catalysis process at the semiconductor–electrolyte interface [18] , [24] . Hence, the significant enhancement of the photocurrent must be due to the LSPR and/or SPP modes in the gold nanohole array. 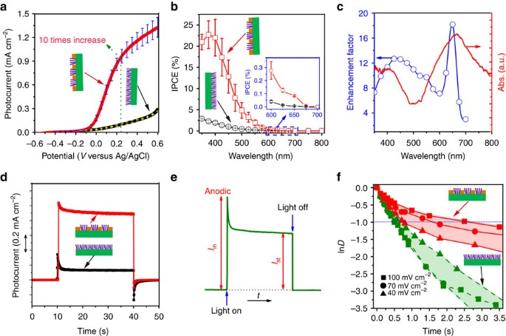Figure 3: Photoelectrochemical performance of the hematite nanorod arrays. (a)J–Vcurves under the illumination of AM 1.5G full-spectrum solar light with a power density of 100 mW cm−2. (b) IPCE spectra; the insert is the IPCE in 600–700 nm range. (c) The photocurrent enhancement factor as a function of the wavelength. (d–f) Anodic photocurrent dynamics of photoelectrodes at an applied bias 0.23 V versus Ag|AgCl. (e) The scheme for the calculation of the transient dynamics is constant. (f) Anodic transient dynamics under AM 1.5G full-spectrum solar light with different irradiation intensities. Error bars are defined by the s.d. over five trials and at least three samples. Figure 3: Photoelectrochemical performance of the hematite nanorod arrays. ( a ) J – V curves under the illumination of AM 1.5G full-spectrum solar light with a power density of 100 mW cm −2 . ( b ) IPCE spectra; the insert is the IPCE in 600–700 nm range. ( c ) The photocurrent enhancement factor as a function of the wavelength. ( d – f ) Anodic photocurrent dynamics of photoelectrodes at an applied bias 0.23 V versus Ag|AgCl. ( e ) The scheme for the calculation of the transient dynamics is constant. ( f ) Anodic transient dynamics under AM 1.5G full-spectrum solar light with different irradiation intensities. Error bars are defined by the s.d. over five trials and at least three samples. Full size image The incident photon-to-electron efficiency (IPCE) spectrum was measured to elucidate the correlation of the LSPR and SPP modes with the enhanced photocurrent ( Fig. 3b ). The hematite nanorods on the Au nanohole pattern showed a substantially enhanced IPCE in the wavelength range from 325 to 700 nm when compared with hematite on bare FTO. The IPCE at 425 nm was 1.37% and 17.4% for the hematite nanorods on the bare FTO and on the long-range ordered Au hole array, respectively. An IPCE enhancement spectrum was obtained by dividing the two corresponding IPCE spectra ( Fig. 3c ), revealing two distinct enhancement peaks of 13 times enhancement at 425 nm and 18 times enhancement at 650 nm. These positions correlate well with the enhanced transmission and absorption of the Au nanohole array, which the finite difference time domain (FDTD) simulations [44] , [45] confirmed as being caused by SPP and LSPR modes, respectively (see Supplementary Fig. S7c ). Charge recombination Charge recombination is typically a large bottleneck in the hematite photoanode. Photocurrent transient measurement was therefore performed to assess whether the metal nanohole array can suppress the charge recombination rate [13] , [14] ( Fig. 3d and Supplementary Fig. S8 ). To quantitatively determine the charge recombination behaviour, a normalized parameter ( D ) is introduced: where I t , I st and I in are the time-dependent, steady-state and initial photocurrent, respectively, as shown in Fig. 3e (ref. 46 ). The transient time constant ( τ ) is defined as the time when lnD =−1 in the normalized plots of lnD − t ( Fig. 3f ), which reflects the general behaviour of charge recombination and lifetime of the charge carriers. τ was estimated to be 2.51 s for the hematite on the long-range ordered Au nanohole array pattern under 100 mW cm −2 of simulated solar light, which was five times that for hematite without the Au nanohole array pattern (0.53 s), indicating the suppressed charge recombination [15] , [47] . The increase in the recombination lifetime was not due to surface chemistry or bulk trapping states, as the onset potential (in Fig. 3a ) did not change with the incorporation of hematite with the plasmonic Au nanohole pattern. Rather, the intense localized electromagnetic (EM) field gradient created by the plasmonic Au nanohole pattern must lead to the lower charge recombination rate. To investigate this effect, the intensity of the incident field was modulated using full-spectrum neutral density filters ( Supplementary Fig. S9 ). The normalized photocurrents demonstrate that the decay was altered when varying the incident light intensity for hematite on the long-range ordered Au nanohole array pattern, whereas no change was observed when varying the light intensity for hematite on the bare FTO. To quantitatively determine these changes in the charge recombination dynamics, the lifetime was measured ( Fig. 3f ). As expected, the lifetime of the carriers increased with an increase in the irradiation intensity for hematite on the long-range ordered Au nanohole array pattern, as the local EM field gradient was proportional to the light intensity. However, hematite on the bare FTO had the same transient time constant within the error scale, independent of the incident intensity, which indicates that the localized EM field near the Au nanoholes must cause a difference in the carrier lifetime. The SPP and LSPR plasmonic fields combine to create an increase in photoconversion efficiency and an increase in carrier lifetime. The different origins of the SPP and LSPR modes, however, lead to two distinct forms of enhancement to the solar energy conversion efficiency, which are complementary across the solar spectrum. In the 300- to 500-nm region, the periodicity of the nanohole array allows the incident light to couple to the SPP mode, which is a travelling charge density wave in the metal film ( Supplementary Fig. S7a ) [37] , [38] , [39] . The travelling SPP mode can re-radiate into the far field when interrupted by a nanohole, increasing the optical transmission at that wavelength ( Supplementary Fig. S7d ) [21] , [38] , [39] , [47] , [48] . As the nanoholes are filled with the hematite nanorods, the increased photon flux from the extraordinary optical transmission will be directly launched into the nanorod instead of being re-radiated from the nanohole. The high contrast in dielectric constant between the semiconductor and the surrounding environment, coupled with the subwavelength nature of the plasmon emission, will therefore allow the SPP to excite a guided mode in the nanorod, increasing absorption in hematite. This behaviour can be seen in a simple FDTD model consisting of a gold nanohole array identical to the one in this experiment but with a single, uniform hematite nanorod grown in each nanohole ( Fig. 4a ). The resulting normalized EM field distribution ( Fig. 4a ) shows that at the SPP resonance (450 nm), the incident light is concentrated in the metal nanohole, which subsequently launches a guided optical mode in the hematite nanorod. The guided nature of the optical mode is revealed by the well-defined nodes in the averaged field ( Fig. 4a ). The mode can be further shown in a cross-cut of the nanowire in Supplementary Fig. S10a,b , which shows that it is distributed mainly in the core of the nanowire but extends into and past the surface as the wavelength increases and the waveguiding efficiency decreases. Even with multiple nanorods in the metal nanohole, waveguiding is still present, creating an optical mode split between each nanorod ( Fig. 4c ). 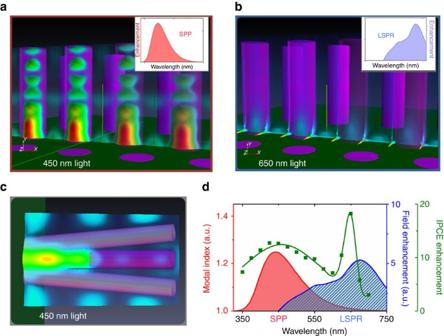Figure 4: FDTD simulations of the Au nanohole array with hematite nanorods. (a) At wavelengths corresponding to an increased transmission in the Au nanohole array, the SPP led to trapping of incident light as waveguided modes in the hematite nanorod. (b) At wavelengths corresponding to the LSPR, no waveguiding is seen, rather the incident field is localized at the edges of the hole. (c) The same waveguiding exists in a simulation more similar to the SEM images ofFig. 1c. (d) The waveguiding efficiency and local field enhancement are seen to accurately explain the experimental IPCE. Figure 4: FDTD simulations of the Au nanohole array with hematite nanorods. ( a ) At wavelengths corresponding to an increased transmission in the Au nanohole array, the SPP led to trapping of incident light as waveguided modes in the hematite nanorod. ( b ) At wavelengths corresponding to the LSPR, no waveguiding is seen, rather the incident field is localized at the edges of the hole. ( c ) The same waveguiding exists in a simulation more similar to the SEM images of Fig. 1c . ( d ) The waveguiding efficiency and local field enhancement are seen to accurately explain the experimental IPCE. Full size image The waveguiding enhancement versus wavelength can be further quantified using mode solver calculations for the realistic, ~120 nm hematite nanorods. The results are displayed in terms of the modal index in Fig. 4d . For the single mode examined, the higher the modal index, the more tightly bound the waveguiding can be thought of as in the hematite core ( Supplementary Fig. S10c ), with a modal index of one corresponding to the absence of waveguiding. The waveguiding efficiency versus the wavelength matches excellently to the 425-nm enhancement peak in the IPCE spectrum ( Fig. 4d ). This confirms that the first enhancement in the IPCE comes from the SPP, which launches a guided optical mode in the nanorod, turning the nanorod into a miniature ‘optical fibre’ and increasing the light absorption at the energies above the band edge of hematite. The SPP leads to an enhanced transmission in the 300- to 500-nm range, whereas the LSPR mode induces an increased absorption in the 550- to 750-nm range ( Supplementary Fig. S7c ). LSPR does not create extraordinary optical transmission. Instead, the absorption of the LSPR creates an intense local field at the walls of the nanohole in the metal film ( Supplementary Fig. S7e ). The energy absorbed by the LSPR can be transferred to the semiconductor at the energies below the band edge through DET [29] , [30] and/or PIRET [31] , allowing an increase in the IPCE. FDTD simulation of the simple model of a uniform hematite nanorod in the metal nanohole array was repeated at the wavelengths close to the LSPR absorption (650 nm). The LSPR created a sharp field enhancement at the metal/hematite interface, but little light was transmitted into the hematite nanorod ( Fig. 4b ). When the peak field enhancement |E/E 0 | 2 was extracted versus the wavelength, it was seen to overlap with the hematite band edge and closely correlate with the second enhancement peak in the IPCE, which confirms that a plasmonic energy-transfer mechanism must be responsible for the enhancement ( Fig. 4d ). In the present work, hematite is not in direct physical contact with the plasmonic Au. DET therefore cannot be responsible for the LSPR-based IPCE enhancement. However, the LSPR absorption band does overlap with the absorption band of hematite, which makes PIRET the most probable plasmonic energy-transfer mechanism [31] . The presence of PIRET was confirmed by conducting similar measurement with a TiO 2 nanorod array on the Au hole array pattern. This control experiment showed no enhancement in the IPCE at 650 nm (data not shown). This is not surprising, because the absorbance band of TiO 2 has no spectral overlap with the LSPR absorbance peak of the Au hole array, which makes PIRET impossible. This confirms that PIRET transfers the energy in the LSPR field to hematite, allowing enhancement in the IPCE at the wavelengths below the band edge of hematite ( Fig. 4d ). The periodicity of the plasmonic pattern can affect the plasmonic properties of the metal nanostructures [49] , [50] . As a control sample, a disordered Au hole array pattern was fabricated with the same hole size but without long-range order ( Supplementary Fig. S11 ). In this disordered hole array, the distance between the holes were varied and dimer and trimer hole pairs existed. The hematite nanorod array was then grown on the disordered Au hole array ( Supplementary Fig. S12 ) and its PEC performance was tested ( Supplementary Fig. S13 ). It can be seen from the ultraviolet–visible absorption spectra ( Supplementary Fig. S5 ) that the SPP transmission peak became weakened and the LSPR peak red-shifted to 800 nm for the disordered Au hole array without hematite nanorods. The red-shift of LSPR peak is due to the coupling between the now-aggregated dimer and trimer hole pairs in the local area ( Supplementary Fig. S14 ). Even though the hole array is highly disordered, a transmission enhancement is still possible due to the periodicity of local disorder domains in the hole array, as shown by FDTD simulation (see Supplementary Fig. S14 and Supplementary Note 1 for detailed analysis). Therefore, the photocurrent of the hematite nanorods array on the disordered Au hole array exhibited only 2.8 times enhancement of that of hematite on the bare FTO substrate at a bias of 0.23 V (versus Ag|AgCl) under the simulated solar full spectrum ( Supplementary Fig. S13a ). The enhancement effect of the disordered Au hole array was smaller than the long-range ordered hole array, which was expected from a decrease in the SPP transmission peak and from the red-shift of the LSPR peak ( Supplementary Fig. S5 ). The disordered hole array allows further confirmation of the separate LSPR- and SPP-based enhancements. It is worth noting that red-shift of the LSPR band ( Supplementary Figs S5 and S14b ) led to no spectral overlap between the absorption edge of hematite and the LSPR absorbance band of the disordered Au hole array, preventing PIRET. The IPCE data reflected this change with no enhancement at the wavelengths above the band edge of hematite ( Supplementary Fig. S13b ). The weak SPP mode in the disordered pattern allowed a small enhancement at the SPP transmission peak (IPCE at 425 nm=5.18%). As the long-range order increases, the SPP transmission becomes stronger and the IPCE enhancement increases in strength but does not change spectrally (comparing Supplementary Fig. S13b with Fig. 3b ). In addition, in the long-range ordered pattern the LSPR band can overlap with the absorption edge of hematite, enabling the PIRET process. By combining SPP and LSPR in a single nanostructure, several new advantages exist when compared with optimization with SPP or LSPR alone [26] , [27] . Not only does the nanohole array launch a confined mode in the nanorods, which should further trap the incident light, it also increases the carrier lifetime due to the plasmonic field. In summary, a broad-wavelength light collection enhancement that spanned the full ultraviolet–near-infrared wavelength range was realized in the hematite nanorod–Au nanohole array pattern architecture. The extraordinary transmission of the SPP modes was used to concentrate the incident light at the energies above the band edge of hematite. The nanorods acted as miniature ‘fibre optics’, creating the confined modes, which trapped the incident light and enhanced the light absorption. The intense local field enhancement of the LSPR overlapped with the absorption band edge of hematite, enhancing solar energy collection at the energies below the band edge through the PIRET mechanism. As a result, the photonic (13 times enhancement at 425 nm) and the plasmonic energy-transfer enhancement (18 times enhancement at 650 nm) were revealed in the IPCE spectrum. Finally, the intense local field gradient increased the carrier lifetime in hematite. This metal/semiconductor heterostructure enhanced both the spectral utilization and the carrier lifetime in the semiconductor in an easy-to-manufacture geometry, making it ideal for plasmon-enhanced solar energy conversion. Synthesis of Au nanohole array pattern The ordered Au nanohole array pattern was fabricated on the FTO substrate with nanosphere lithography [40] , [42] . The FTO substrate was first treated with the acid solution to have a hydrophilic surface. Next, 500-nm-sized polystyrene (PS) monolayer was assembled on the FTO substrate. A 5-nm thick Ti, 45-nm thick Au, 5-nm thick Ti and 30-nm thick SiO 2 layer were subsequently deposited on the FTO surface in sequence with an e-beam evaporation. Finally, the nanohole array pattern was obtained after lift-off of the PS spheres. For the disordered Au nanohole array, the same procedure was employed, except that the PS template was dispersed on the FTO substrate by spin-coating instead of self-assembly on the water surface. Growth of hematite nanorod array Following a low-temperature hydrothermal method [43] , the hematite nanorod array was grown on the bare FTO and on the Au hole array pattern, respectively. Briefly, 0.15 M FeCl 3 and 1 M NaNO 3 were dissolved in 40 ml of deionized water. Concentrated HCl was dropped into the solution to adjust the pH value to ~1.5. Precleaned FTO and the Au nanohole array substrates were placed into a Teflon-lined autoclave. The autoclave was heated at 100 °C for different growth times to obtain different lengths of hematite nanorods. After completing washing with deionized water and ethanol, the hematite nanorods were annealed in air at 650 °C for 20 min. Characterization The morphology of the hematite nanorods and the Au nanohole array pattern were observed with a field-emission scanning electron microscope (JEOL 7600F) and a TEM (JEOL JEM 2100F), respectively. The crystal structure of hematite nanorods was characterized with a high-resolution TEM (JEOL JEM 2100F) and X-ray diffraction (X′ Pert Pro PW 3040-Pro, Panalytical Inc.) with Cu K α radiation. The light-absorption properties were measured by the diffuse-reflection mode with Shimadzu 2550 ultraviolet–visible spectrometer equipped with an integrating sphere (UV 2401/2, Shimadzu). Absorption measurement was taken using an integrating sphere to reduce the effects of scattering of the nanorod array on the measurement. Both transmission and reflection were measured to calculate the absorption. Photoelectrochemical measurement The PEC behaviour of hematite was tested with a three-electrode configuration with a Gamry Reference 3000 Potentiostat/Galvanostat/ZRA instrument. The hematite nanorod array was employed as the working electrode, the Pt foil as the counter electrode and Ag|AgCl as the reference electrode. NaOH (1 M) aqueous solution was used as an electrolyte and bubbled with N 2 for 30 min before measurement. The light source employed in this study was a 300-W Xenon lamp with an AM 1.5G filter. All the PEC measurements were performed on at least three samples and each sample was tested at least three times. The spectra of IPCE were measured by the same light source coupled with a monochromator (Oriel Cornerstone 130, 1/8 cm). IPCE can be expressed as [16] where J is the measured photocurrent density (mA cm −2 ), λ is the wavelength of the incident light (nm) and I light is the measured irradiance at the specific measurement wavelength (W m −2 ). FDTD simulations To confirm the origin of the enhancement observed in the IPCE spectrum, FDTD simulations were run using the commercially available Optiwave software, similar to our previous work [44] , [45] . The mode calculations were performed using Optimode. The simulation cell was constructed identically to the Au nanohole array ( Fig. 1a ) and the corresponding ultraviolet–visible spectrum was matched to that of the Au nanohole array ( Fig. 2a ) to ensure consistency ( Fig. 4c ). The hematite was modelled using the full frequency-dependent dielectric function [51] , Au and titanium using the data of Palik [52] and SiO 2 using a refractive index of 1.4. The reported values of bulk Fe 2 O 3 vary depending on the synthesis procedure [53] . For the simulation, an absorption coefficient of 5 × 10 4 at 500 nm was used. The resolution of the cell was 2 nm and the input wave was a Gaussian pulse, linearly polarized in the y direction. Periodic boundary conditions were used to replicate the periodic nanohole array. The local field was examined versus the excitation wavelength to confirm the nature of the plasmonic modes. The local field was normalized by that in the absence of the nanostructure and was reported as |E/E 0 | 2 . The local field of the LSPR mode was determined by measuring the maximum at each excitation wavelength. If multiple maximums were present at different locations, the largest field enhancement was reported. A field enhancement was present at both SPP and LSPR modes. However, in the SPP, the field enhancement led to an increased transmission, masking the maximum field enhancement. Therefore, the field enhancement was only reported in the region of the LSPR where increased transmission was negligible. Identification of SPP and LSPR modes Two modes can exist in the metal nanohole array. The first is SPP, which corresponds to an oscillating charge wave at the metal–semiconductor interface ( Supplementary Fig. S7a ). The SPP can only be excited by matching the momentum of the charge wave to the incident photon through the periodicity of the nanostructure. Just as the periodicity allows coupling to incident light, the SPP modes can recouple to the far field on the opposite side of the nanohole array, leading to an enhanced transmission ( Supplementary Fig. S7d ). The LSPR does not propagate and, instead, is localized at the edges of the nanohole. The local charge oscillations lead to an intense local field at the interfaces of the metal/dielectric ( Supplementary Fig. S7e ). In the LSPR, the momentum matching comes from the curvature of the nanoscale shape and is only dependent on the geometry of the nanohole and not on the periodicity of the array. Therefore, an increase in absorption or transmission can easily be assigned to a SPP or LSPR mode by turning off the periodicity in the FDTD boundary conditions ( Supplementary Fig. S7c ). How to cite this article: Li, J. et al . Plasmon-induced photonic and energy-transfer enhancement of solar water splitting by a hematite nanorod array. Nat. Commun. 4:2651 doi: 10.1038/ncomms3651 (2013).